Globally homochiral assembly of two-dimensional molecular networks triggered by co-absorbers Understanding the chirality induction and amplification processes, and the construction of globally homochiral surfaces, represent essential challenges in surface chirality studies. Here we report the induction of global homochirality in two-dimensional enantiomorphous networks of achiral molecules via co-assembly with chiral co-absorbers. The scanning tunnelling microscopy investigations and molecular mechanics simulations demonstrate that the point chirality of the co-absorbers transfers to organizational chirality of the assembly units via enantioselective supramolecular interactions, and is then hierarchically amplified to the global homochirality of two-dimensional networks. The global homochirality of the network assembly shows nonlinear dependence on the enantiomeric excess of chiral co-absorber in the solution phase, demonstrating, for the first time, the validation of the ‘majority rules’ for the homochirality control of achiral molecules at the liquid/solid interface. Such an induction and nonlinear chirality amplification effect promises a new approach towards two-dimensional homochirality control and may reveal important insights into asymmetric heterogeneous catalysis, chiral separation and chiral crystallization. Two-dimensional (2D) chirality of molecular self-assembly on solid surfaces has gained wide spread interest because of its fundamental significance and potential applications. Mechanistic studies of the induction, transformation and amplification of chirality on 2D surfaces grant fundamental understanding of enantioselective heterogeneous catalysis, chiral separation, chiroptical materials and sensors, and may provide insights into the origin of chirality in biomolecules and life [1] , [2] , [3] , [4] , [5] , [6] , [7] , [8] , [9] . Through the adsorption of chiral molecules, 2D chirality can be endowed to achiral solid surfaces [10] , [11] , [12] . Besides, self-assembly of achiral molecules on achiral surfaces could induce 2D chirality due to reduced freedom and the constraint of the substrate lattice [13] , [14] , [15] , [16] . However, the spontaneous resolution of achiral molecules into 2D enantiomorphous assemblies shows no chiral bias and typically leads to globally racemic surfaces. Developing efficient routes to control the chirality of 2D molecular assembly and obtain globally homochiral surfaces represents an essential challenge in 2D chirality studies. In analogy to the chirality amplification in 1D helical covalent and supramolecular polymeric systems, the so-called sergeants-and-soldiers principle and the majority rules have been applied to tailor 2D homochirality [17] , [18] , [19] , [20] , [21] , [22] , [23] , [24] , [25] . For the former, chirality control is achieved via co-deposition of a few chiral molecules as chiral inducers with the achiral molecules [26] , [27] , [28] , [29] . The representative study is the induction of homochiral assembly of achiral succinic acid (SU) on Cu(110) by co-deposition of tartaric acid (TA) enantiomer, in which a few ‘TA sergeants’ serve as chiral seeds and force adjacent ‘SU soldiers’ adopting the same absolute configuration. It is reported that 2 mol% of chiral TA is sufficient to completely suppress the chirality opposite SU enantiomorph and induce homochirality on the surface [28] . On the basis of this principle, the induction of homochirality in achiral enantiomorphous monolayers by elaborately designing and synthesizing chiral sergeants with similar structure to the achiral molecules has been demonstrated [26] , [27] . As for the majority rules, they refer to a nonlinear dependence of chiral supramolecular assembly on the enatiomeric excess (ee) of the chiral monomers. Ernst and co-workers [30] reported that a small excess of one of the heptahelicene enantiomers is enough to construct homochiral surfaces consisting of domains with only one of two possible lattice structures. Similarly, a homochiral adlayer of TA is achieved via introducing a small enantiomeric imbalance of two enantiomers [31] . However, the nonlinear chirality amplification in molecular assemblies on solid surfaces consisting of achiral molecules has not been demonstrated. In addition, few examples have shown that 2D homochirality can be achieved by external means such as magnetic field and chiral solvent [32] , [33] , [34] , [35] , [36] . For example, De Feyter et al. have shown that the formation of 2D molecular rosettes can be biased towards being either right-handed or left-handed by using a chiral solvent [36] . Herein, we demonstrate the induction and nonlinear amplification of homochirality in an enantiomorphous 2D assembly of an achiral molecule tailored by co-assembly with a chiral co-absorber at the liquid/solid interface. The enantiomorphous porous networks of 5-(benzyloxy)-isophthalic acid derivative (BIC) on highly oriented pyrolytic graphite (HOPG) surface show global homochirality upon co-deposition of enantiopure chiral 2-octanol. The point chirality of the co-absorber is transferred to organization chirality through supramolecular hydrogen bonding interactions, which is then hierarchically amplified to 2D assembly with global homochirality. Intriguingly, global homochirality of the assembled networks can be realized when the excess of one enantiomer of 2-octanol reaches ≥5.2%, illustrating a nonlinear chirality amplification. To the best of our knowledge, it is the first time to demonstrate the majority rules applicability in 2D molecular assemblies from achiral molecules. The global homochirality can be memorized by site replacement of 2-octanol with other achiral co-absorbers. This result paves a simple and efficient strategy to control the global homochirality of 2D molecular assemblies. It also provides important insights into the induction and amplification of chirality in 2D surfaces, which are pertinent to many important chemical processes, such as asymmetric heterogeneous catalysis, chiral separation and enantioenrichment in crystal chemistry. 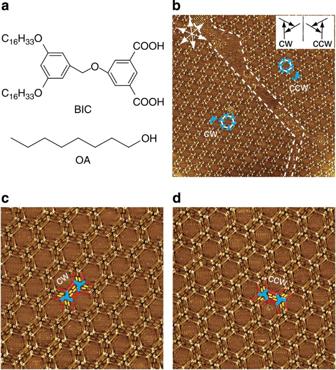Figure 1: Self-assemblies of BIC at the OA/HOPG interfaces. (a) Chemical structures of BIC and OA. (b) Large-scale STM image (93 × 93 nm2,I=0.205 nA,Vbias=0.900 V) of BIC monolayer at the OA/HOPG interface. The dotted lines indicate domain boundaries. The white hexagons indicate the hexagonal units in BIC assembly. The blue windmills and arrows indicate the BIC trimers and their rotational directions, respectively. The white arrows indicate the substrate lattice of HOPG. Inset, CW and CCW rotation of a BIC trimer is defined by the vectors from the benzene ring attached with the alkoxy chains to the isophthalic acid moiety. (c) High-resolution STM image (38 × 38 nm2,I=0.066 nA,Vbias=0.912 V) of the CW network. (d) High-resolution STM image (40 × 40 nm2,I=0.065 nA,Vbias=0.900 V) of the CCW network. The blue, red and yellow lines incanddoutline the bright aromatic cores, the alkoxy chains in BIC, and the alkyl chains in the solvent, respectively. Enantiomorphous nanoporous networks Figure 1a shows the chemical structures of BIC molecule and 1-octanol (OA). BIC possesses an aromatic core, equipped with two carboxylic acid functional groups on one side, and two alkoxy chains on the other side. BIC forms well-defined hexagonal porous networks at the OA/HOPG interface with a concentration of 1 × 10 −5 M, as shown in Fig. 1b . The unit cell parameters are measured to be a = b =6.8±0.1 nm and α =60±1°. Each vertex of the hexagon is composed of three bright rods arranged in a rotary manner. Considering the molecular structure and the scanning tunnelling microscopy (STM) image, the bright rods are assigned to the aromatic cores of BIC molecules. Careful inspection reveals that two kinds of molecular trimers form in the BIC assembly; one rotates clockwise (CW), whereas the other rotates counterclockwise (CCW), as schematically shown in the inset of Fig. 1b . Molecular trimers with the same handedness further assemble into homochiral domains. The domains consisted of CW trimers and those composed of CCW trimers are enantiomers to each other, which are defined as CW and CCW networks, respectively. As expected, the CW and CCW domains present with no bias on the substrate, rendering the entire surface globally racemic. Figure 1: Self-assemblies of BIC at the OA/HOPG interfaces. ( a ) Chemical structures of BIC and OA. ( b ) Large-scale STM image (93 × 93 nm 2 , I =0.205 nA, V bias =0.900 V) of BIC monolayer at the OA/HOPG interface. The dotted lines indicate domain boundaries. The white hexagons indicate the hexagonal units in BIC assembly. The blue windmills and arrows indicate the BIC trimers and their rotational directions, respectively. The white arrows indicate the substrate lattice of HOPG. Inset, CW and CCW rotation of a BIC trimer is defined by the vectors from the benzene ring attached with the alkoxy chains to the isophthalic acid moiety. ( c ) High-resolution STM image (38 × 38 nm 2 , I =0.066 nA, V bias =0.912 V) of the CW network. ( d ) High-resolution STM image (40 × 40 nm 2 , I =0.065 nA, V bias =0.900 V) of the CCW network. The blue, red and yellow lines in c and d outline the bright aromatic cores, the alkoxy chains in BIC, and the alkyl chains in the solvent, respectively. Full size image STM images of the BIC assembly at the OA/HOPG interface with higher resolution are shown in Fig. 1c . It is revealed that the vertexes of the hexagons are occupied by the chiral molecular trimers, which are bridged by the paralleled alkoxy chains with depressed contrast. These alkyl chains can be divided into two groups: longer alkyl chains located at the brim of the bridges and shorter alkyl chains between the longer alkyl chains, illustrated with red and yellow sticks, respectively. The former corresponds to the interdigitated alkoxy chains in BIC molecules, and the latter are ascribed to co-adsorbed OA molecules, after considering the dimension of the STM features. Four co-adsorbed OA molecules are found between two chiral molecular trimers. Thus, the ratio between BIC and the co-absorbers is 1:2 in the assembly. Control of global homochirality by chiral co-absorber When the achiral OA is changed to chiral (R)-(−)-2-octanol (R-OA), a similar honeycomb network is obtained ( Fig. 2a ). The unit cell parameters and structural features in the assembly are the same as those for the assembly at the OA/HOPG interface. Statistical analysis of over 200 images collected at different locations and different batch of samples reveals all domains show the same CW handedness, indicating that a globally homochiral porous network is obtained at the R-OA/HOPG interface. For comparison, we investigated the co-assembly of BIC and (S)-(−)-2-octanol (S-OA) under the same experimental conditions. Intriguingly, only CCW domains are observed, and no CW structure is formed ( Fig. 2b ). These results indicate that by co-depositing chiral 2-octanol, the handedness of the 2D enantiomorphous networks of BIC at the liquid/solid interface can be controlled, with 100% of the assembly showing the same handedness. 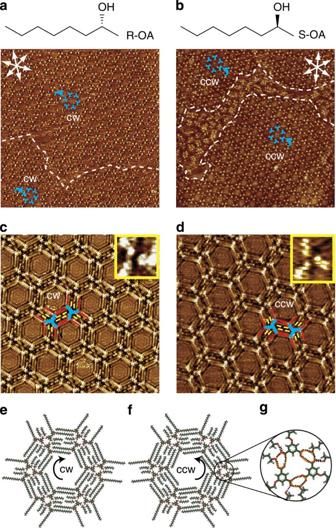Figure 2: Self-assemblies of BIC at the chiral 2-octanol/HOPG interfaces. (a) Large-scale STM image (100 × 100 nm2,I=0.205 nA,Vbias=0.900 V) of BIC at R-OA/HOPG interface. (b) Large-scale STM image (100 × 100 nm2,I=0.100 nA,Vbias=0.900 V) of BIC at S-OA/HOPG interface. The dotted lines indicate domain boundaries. The blue windmills and arrows indicate the BIC trimers and their rotational directions, respectively. The white arrows indicate the substrate lattice directions of HOPG. (c) High-resolution STM image (30 × 30 nm2,I=0.095 nA,Vbias=0.929 V) of BIC monolayer at R-OA/HOPG interface. (d) High-resolution STM image (30 × 30 nm2,I=0.100nA;Vbias=0.900 V) of BIC monolayer at S-OA/HOPG interface. Inset: zoom-in images of single BIC trimers. The blue, red and yellow lines outline the bright aromatic cores, the alkoxy chains in BIC and the alkyl chains in solvent, respectively. (e) Structural model of CW network at R-OA/HOPG interface. (f) Structural model of CCW network at S-OA/HOPG interface. (g) Illustration of the intermolecular interactions within the molecular trimer. The black dotted lines represent the intermolecular hydrogen bonds. The orange circle indicates the 10-member ring formed by two carboxylic acid groups in neighboring BIC molecules and a hydroxyl group in the solvent molecule, connecting by three O-H…O hydrogen bonds. Figure 2: Self-assemblies of BIC at the chiral 2-octanol/HOPG interfaces. ( a ) Large-scale STM image (100 × 100 nm 2 , I =0.205 nA, V bias =0.900 V) of BIC at R-OA/HOPG interface. ( b ) Large-scale STM image (100 × 100 nm 2 , I =0.100 nA, V bias =0.900 V) of BIC at S-OA/HOPG interface. The dotted lines indicate domain boundaries. The blue windmills and arrows indicate the BIC trimers and their rotational directions, respectively. The white arrows indicate the substrate lattice directions of HOPG. ( c ) High-resolution STM image (30 × 30 nm 2 , I =0.095 nA, V bias =0.929 V) of BIC monolayer at R-OA/HOPG interface. ( d ) High-resolution STM image (30 × 30 nm 2 , I =0.100nA; V bias =0.900 V) of BIC monolayer at S-OA/HOPG interface. Inset: zoom-in images of single BIC trimers. The blue, red and yellow lines outline the bright aromatic cores, the alkoxy chains in BIC and the alkyl chains in solvent, respectively. ( e ) Structural model of CW network at R-OA/HOPG interface. ( f ) Structural model of CCW network at S-OA/HOPG interface. ( g ) Illustration of the intermolecular interactions within the molecular trimer. The black dotted lines represent the intermolecular hydrogen bonds. The orange circle indicates the 10-member ring formed by two carboxylic acid groups in neighboring BIC molecules and a hydroxyl group in the solvent molecule, connecting by three O-H…O hydrogen bonds. Full size image High-resolution STM images are scrutinized to get insights into the origin of the remarkable bias for the formation of globally homochiral networks. Figure 2c are the high-resolution STM images of the CW and CCW patterns formed at the R-OA/HOPG and S-OA/HOPG interfaces, respectively. It is revealed that the chiral 2-octanol molecules are also involved in the assembly of BIC. Four 2-octanol molecules are entrapped in the barrier enclosed by neighbouring BIC trimers. On the basis of these results, structural models of the CW and CCW patterns are proposed, as shown in Fig. 2e . At the node of the nanoporous network, every three BIC molecules form a supramolecular trimer via hydrogen bonding between carboxylic acid groups. The leftover hydrogen bonding sites are saturated by the hydroxyl end of the octanol molecule (OA, R-OA or S-OA). Figure 2g reveals the details of the hydrogen bonding at the vertex of the hexagon. Three hydrogen bonds are formed between neighbouring BIC molecules in the trimer. The OH group from one 2-octanol molecule takes part in a 10-member ring, stabilized by three O-H…O hydrogen bonds, as outlined by the orange circles in Fig. 2g . Another 2-octanol molecule attaches to the 10-member ring to saturate the hydrogen bonding acceptor of BIC. The structural models are consistent with the molecular ratio and structural features observed in the STM images. Diluting the chiral 2-octanol in the solution with an inert solvent, such as 1-octylbenzene (OB), does not change the ability of chiral 2-octanol to induce the chiral assembly of BIC. In fact, a globally homochiral BIC assembly can be obtained when the concentration of chiral co-absorber in the solution phase is as low as 10% (volume ratio) ( Supplementary Fig. S1 ). Further decreasing of the concentration of 2-octanol in OB results in the formation of square assemblies of BIC, presumably due to the change of solution concentration and polarity [37] . In contrast, the enantiomeric bias for the formation of a globally homo chiral assembly of BIC is lost when using a mixed solvent of achiral OA and chiral R-OA (or S-OA). The STM results show that the CW and CCW networks coexist in the monolayer even when 90% of the mixed solvent is R-OA (or S-OA). Statistics results reveal that 53±7% of the area of the networks show CCW handedness, suggesting no bias for CW and CCW networks. The result implies that the assembly of BIC in the mixed solution of achiral OA and chiral 2-octanol may be dominated by achiral component OA. The molecular mechanics (MM) calculation further supports that the stability of BIC nanoporous networks with co-adsorbed OA is higher than that with co-adsorbed chiral R-OA or S-OA ( Table 1 ). Table 1 Relative total energies from MM simulations of the BIC trimers and hexagonal units binding with different co-absorbers. Full size table Majority rules at the liquid/solid interface The observation of global homochiral assembly of BIC in the presence of enantiopure 2-octanol co-absorber promotes us to investigate the assemblies of BIC in the presence of both R-OA and S-OA with different ratios. Statistical analysis indicates that CW network and CCW network coexist with equal percentage in the assembly when R-OA:S-OA in the mixed solvent is 1:1. Once an enantiomeric unbalanced mixed solution is used, bias for the network enantiomorph emerges. 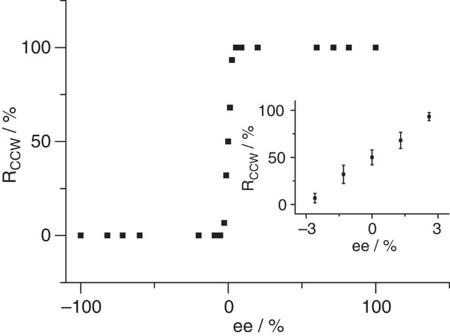Figure 3: Nonlinear amplification of homochirality in BIC assembly. Area percentage of CCW network in the monolayer as a function of the excess of S-OA in the mixture of R-OA and S-OA shows typical S-shape nonlinear behaviour, which indicates that the majority rules are operative. ee is defined as ee=(NS−NR)/(NS+NR), in whichNSandNRare the amount of S-OA and R-OA in the mixed solvents, respectively.RCCWis the area percentage of CCW network in the assembly. Inset is a magnified curve with error bars, which reveal the s.d. of several studied samples. Figure 3 shows the area percentage of the CCW network within the monolayer ( R CCW ) as a function of the excess of S-OA. A typical S-shape nonlinear behaviour of the R CCW to ee of S-OA evolves, which indicates the so-called majority rules dominate the formation of the porous network [38] , [39] . As is shown, when the ee of S-OA is 1.3%, 68±8% of the area of the assembly are CCW. When the ee of S-OA increases to 2.6%, the R CCW reaches 93±12%. Once the excess of S-OA is ≥5.2% (S-OA:R-OA=10:9), all domains in the monolayer are CCW. Similarly, when an excess of R-OA reaches ≥5.2% (S-OA:R-OA=9:10), 100% enantiomeric bias of the CW-assembled networks occurs ( Fig. 3 ). The critical ee for achieving global homochiral assemblies in the present system is lower than that for the 2D assemblies of heptahelicene and TA, which is 8% and 20%, respectively [30] , [31] . We emphasize that the majority rules are observed only for chiral molecules assembled on surfaces under ultrahigh vacuum conditions in those previous studies. The nonlinear dependence of the 2D chiral assembly of achiral BIC molecules to the ee of co-adsorbed 2-octanol indicates the majority rules are valid for the 2D supramolecular assembly of achiral molecules at liquid/solid interfaces. Figure 3: Nonlinear amplification of homochirality in BIC assembly. Area percentage of CCW network in the monolayer as a function of the excess of S-OA in the mixture of R-OA and S-OA shows typical S-shape nonlinear behaviour, which indicates that the majority rules are operative. ee is defined as ee=( N S − N R )/( N S + N R ), in which N S and N R are the amount of S-OA and R-OA in the mixed solvents, respectively. R CCW is the area percentage of CCW network in the assembly. Inset is a magnified curve with error bars, which reveal the s.d. of several studied samples. Full size image Next, we probe whether the majority rules are still operative when the chiral co-absorber is diluted by an inert solvent. In these measurements, 1 × 10 −5 M BIC is dissolved in the mixed solvent of S-OA, R-OA and OB. It is found that the majority rules effect depends on the ee of the 2-octanol enantiomer as well as on the fraction of 2-octanol in the solution ( C OA =( N S + N R )/( N S + N R + N OB ), N OB is the volume of OB). When ee=5.2%, the majority rules are effective until the disappearance of the porous networks ( C OA ≤10%). However, at ee=2.6%, the bias for the formation of enantiomeric networks diminishes quickly ( R cw changes from 93±12% to 62±6.8% when C OA decreases from 100% to 50%), implying the critical ee for the majority rules effect is lowered upon dilution. (see Supplementary Table S1 for details). Homochiral surfaces with achiral molecules Once a surface assembly with global homochirality is achieved, we try to replace the chiral co-absorber 2-octanol molecules with other achiral molecules. After determination of globally homochiral CW (or CCW) networks at the R-OA/HOPG (or S-OA/HOPG) interface, 0.5 μl of 1,16-hexadecanediol dissolved in R-OA (or S-OA) was added to the liquid/solid interface. Then, the sample was again imaged by STM. It is found that the assembly did not change in 4 h after the addition of 1,16-hexadecanediol. After 4 h, chiral 2-octanol molecules, co-adsorbed in the assemblies, are replaced by 1,16-hexadecanediol molecules. 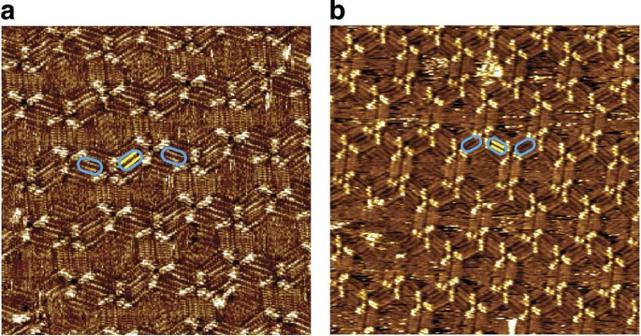Figure 4: Replacement of chiral 2-octanol with achiral 1,16-hexadecanediol. (a) STM image (30 × 30 nm2,I=0.120 nA;Vbias=0.900 V) of the CW network after replacing R-OA with 1,16-hexadecanediol. (b) STM image (40 × 40 nm2,I=0.117 nA;Vbias=0.900 V) of the CCW network after replacing S-OA with 1,16-hexadecanediol. The blue frames highlight that two longer chains instead of four shorter 2-octanol molecules are entrapped. The yellow lines are used to represent the 1,16-hexadecanediol molecules. Figure 4 shows typical STM images after the replacement of chiral 2-octanol molecules by 1,16-hexadecanediol molecules. Molecules entrapped in the barrier enclosed by neighbouring BIC trimers are two longer chains instead of four shorter chains, suggesting that chiral co-adsorbed 2-octanol have been replaced by achiral 1,16-hexadecanediol. At the same time, the global homochirality is sustained. Therefore, a globally homochiral surface with exclusively achiral component is obtained [29] . It is suspected that during the volatilization of chiral 2-octanol, the concentration of 1,16-hexadecanediol at the liquid/solid interface increases step by step. Moreover, the binding energy of 1,16-hexadecanediol is higher than that of 2-octanol. Thus, 1,16-hexadecanediol can replace 2-octanol and give a homochiral assembly composed exclusively of achiral components. The homochiral networks with BIC and 1,16-hexadecanediol can be observed at the air/HOPG interface 24 h after placing the sample in air. The perfect memorization effect further supports high stability of the 2D self-assembled nanoporous network and hints at the potential of so-obtained homochiral networks for chiral resolution and recognition of other species. Figure 4: Replacement of chiral 2-octanol with achiral 1,16-hexadecanediol. ( a ) STM image (30 × 30 nm 2 , I =0.120 nA; V bias =0.900 V) of the CW network after replacing R-OA with 1,16-hexadecanediol. ( b ) STM image (40 × 40 nm 2 , I =0.117 nA; V bias =0.900 V) of the CCW network after replacing S-OA with 1,16-hexadecanediol. The blue frames highlight that two longer chains instead of four shorter 2-octanol molecules are entrapped. The yellow lines are used to represent the 1,16-hexadecanediol molecules. Full size image MM simulations We perform MM simulations to get thermodynamic insight into the chiral co-absorber-induced globally homochiral surface. The relative energies of the CW and CCW trimers and hexagonal units combined with OA, R-OA or S-OA are listed in Table 1 (See Supplementary Figs S2 and S3 for the optimized triangular and hexagonal units from MM simulations). The energy of the CW/OA trimer unit is nearly the same as that of the CCW/OA trimer unit, implying comparable stability of CW/OA and CCW/OA trimer units. The simulation result is consistent with the coexistence of CW/OA and CCW/OA trimer units in the BIC assemblies at the OA/HOPG interface, as revealed by STM results. When achiral OA is changed to chiral R-OA or S-OA, energy bias for one of two enantiomeric trimer units is obtained. The energy of the CW/R-OA trimer unit is close to that of its enantiomeric CCW/S-OA trimer unit, which is about 13.1 kcal mol −1 (4.3 kcal mol −1 per OA pair) higher than the energy of their diastereomic CCW/R-OA and CW/S-OA trimer units. These results indicate that the CW/R-OA and CCW/S-OA trimer units are much more stable than the CCW/R-OA and CW/S-OA trimer units, which explain the selective formation of CW/CCW enantiomeric trimer units in the presence of R-OA or S-OA. Moreover, the energy difference between the CW/R-OA and CCW/R-OA (or between the CCW/S-OA and CW/S-OA) combinations further amplified when the homochirality extends to larger hexagonal units. As shown in Table 1 , the energy difference between the CW/R-OA (or CCW/S-OA) hexagonal unit and the CCW/R-OA (or CW/S-OA) hexagonal unit reaches ca. 90 kcal mol −1 (5.0 kcal mol −1 per OA pair). It is noted that the relative energies of the CW and CCW trimer units co-adsorbed with OA is ~27.4 kcal mol −1 (9.1 kcal mol −1 per OA pair) lower than that with R-OA or S-OA. Therefore, the co-adsorption of OA with BIC molecules is dominated in the presence of both achiral OA and chiral R-OA (or S-OA). The theoretical results can account for the coexistence of CW and CCW domains when a mixed solution of achiral OA and chiral R-OA (S-OA) is used. The induction and propagation of homochirality are two key processes for the formation of globally homochiral structures. In the present study, the induction of single-handed assemblies is attributed to the stereoselective interactions between the chiral co-absorber and BIC trimers. As shown in Fig. 5a , three hydrogen bonds form between BIC molecules within the trimer. The flip of carboxylic acid, which easily occurs in solution, is prohibited in 2D assemblies as the process can significantly rupture the hydrogen bonding among BIC in the trimers. The directional hydrogen bonds within molecular trimers make the BIC molecules arrange in a chiral manner. Two mirror spiral arranged supramolecular trimers, that is, CW and CCW, can be formed by BIC. Accordingly, the leftover hydrogen bonding sites in BIC trimers arrange in a chiral manner too. For example, the –C=O groups are located at the left/right side of the –OH groups in the CW/CCW trimers. The left over hydrogen bonding sites in BIC trimers enclose three chiral hydrogen bonding pockets (marked with blue and green arrows pointing from –OH group to –C=O group in Fig. 5a ). Specific complementary geometry that fits exactly to the pocket is required for the guest molecule to interact with the pockets. We note that a –OH group fits this chiral hydrogen bonding pocket. It can form three effective hydrogen bonds with one such chiral hydrogen bonding pocket and switch on the 10-member ring. For OA molecules, two mirror conformers (named δ-OA and γ-OA) exist upon adsorption on the HOPG surface. The position and direction of the –OH group in the δ-OA and γ-OA conformers match very well with the chiral pockets in CW and CCW trimers, respectively, as shown in Fig. 5a . One OA molecule is entrapped in the pocket and form two hydrogen bonds with the BIC trimer; another OA molecule saturates the other hydrogen bonding site of the pocket. As for chiral R-OA, the molecular conformer with methyl group pointing out of the surface is preferred due to the steric hindrance effect, as revealed by MM simulations. As a result, the –OH group in the adsorbed R-OA molecule is pointed to the left side of the alkyl chains, as determined by the chiral centre. This conformer perfectly fits the host chiral pocket in the CW BIC trimer. It can form two effective O-H…O hydrogen bonds with the pocket in the CW BIC trimer and switch on the 10-member ring. The other hydrogen bonding site of the pocket is saturated by another R-OA molecule. In contrast, the conformation of the adsorbed R-OA molecule does not match the interaction sites of the pocket in the CCW trimer ( Supplementary Fig. S2 ). In fact, S-OA molecules show specific recognition to the CCW BIC trimer. That is, R-OA (or S-OA) shows enantioselective interactions to the CW (or CCW) BIC trimers. Through that, the point chirality of R-OA (or S-OA) is transferred to the CW/R-OA (or CCW/S-OA) trimer aggregations and induces homochirality to the assembly. Exact fit of the geometric shapes as well as the interactional ways is required and responsible for the induction of the homochirality. Our attempt to use other hydrogen bond donors, such as carboxylic acid, to construct a similar nanoporous network failed. This control experiment further illustrates the importance of a close fit of the chiral co-absorber and the chiral pocket in the BIC trimer in the homochiral surface formation. 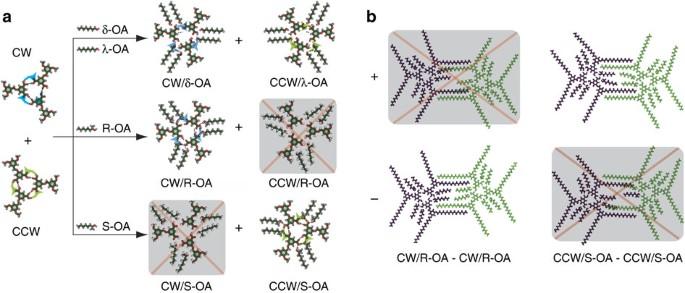Figure 5: Induction and amplification of homochiralityviaspecific recognition between BIC trimer and octanol. (a) Illustration of the induction of homochirality. The alkoxy chains in BIC are replaced by methoxy groups for simplicity. The blue and green arrows indicate the direction of the chiral pockets formed by the leftover hydrogen bonding sites in the BIC trimers, which point from the –OH group to the –C=O group. The red crosses indicate that the units are unstable. (b) Possible interdigitation modes of the neighouring trimer units at the R-OA/HOPG and S-OA/HOPG interface. The trimer units are coloured for identification. The red crosses represent the structures that are unfavoured. Figure 5: Induction and amplification of homochirality via specific recognition between BIC trimer and octanol. ( a ) Illustration of the induction of homochirality. The alkoxy chains in BIC are replaced by methoxy groups for simplicity. The blue and green arrows indicate the direction of the chiral pockets formed by the leftover hydrogen bonding sites in the BIC trimers, which point from the –OH group to the –C=O group. The red crosses indicate that the units are unstable. ( b ) Possible interdigitation modes of the neighouring trimer units at the R-OA/HOPG and S-OA/HOPG interface. The trimer units are coloured for identification. The red crosses represent the structures that are unfavoured. Full size image It is supposed that the interactions between 2-octanol molecules weakly adsorbed in the hexagonal pores or diffused in the liquid phase and the BIC networks may have a less crucial role in the induction of homochirality. First, 10.0% S-OA in a mixed solvent of S-OA and OB is enough to control the homochirality of BIC assembly, implying that a large amount of chiral 2-octanol molecules is not indispensable for the induction of homochirality. Second, the coexistence of CW and CCW domains is observed in the presence of both achiral OA and chiral R-OA (or S-OA). According to MM simulations, the relative energies of the CW and CCW trimer units co-adsorbed with OA is ~27.4 kcal mol −1 (9.1 kcal mol −1 per OA pair) lower than that with R-OA or S-OA. Thus, in the mixture of OA and S-OA or R-OA, OA molecules are preferentially adsorbed on the substrate and result in a monolayer composed of CW and CCW networks with nearly equal percentage. The result indicates that the molecules co-adsorbed with BIC (achiral OA) rather than those in the solution phase (chiral R-OA or S-OA) are important to induce the surface homochirality. Third, we performed MM calculations on BIC hexagonal units with several R-OA or S-OA entrapped in the pores and found that chiral enantiomer of R-OA or S-OA shows no energy bias to favour one of the chiral BIC hexagonal pores. Finally, the formation of global homochirality assembly of BIC is supposed to be related to the strong supramolecular interactions between BIC aggregates and chiral 2-octanol, as well as the participation of the co-absorber in the assembly process. De Feyter’s group reported the chiral solvent and chiral auxiliary-biased formation of 2D enantiomeric assembly of achiral molecules [29] , [36] , although with relatively low ee. Coincidently, the chiral solvent or chiral auxiliary is not indispensible for the formation of the assembly. In the present work, although chiral 2-octanol is used as the solvent, it takes part in the assembly as co-absorber and dictates the organization chirality via enantioselective supramolecular interactions. Therefore, either no hexagonal network forms or all the formed hexagonal networks possess the same handedness. The chirality of BIC trimer units is further transferred and propagated through a hierarchical supramolecular self-assembly process to 2D surface. As shown in Fig. 2 , the alkoxyl chains in the neighbouring BIC trimers interdigitate to each other and form a honeycomb network. There are two possible interdigitation modes: the alkoxyl chains in the left BIC molecular trimer are at the top (+ interdigitation mode) or at the bottom (− interdigitation mode). Therefore, there are four interdigitation motifs for neighbouring BIC trimers in OA, as shown in Supplementary Fig. S4 . First, interdigitation motifs in which neighbouring BIC trimers have opposite handedness are unstable as some of the alkoxyl chains in BIC molecules either overlap or are too close to the alkyl chains of the co-adsorbed OA molecules. Then, the neighbouring alkoxyl chains in the+(or −) interdigitation pattern is undesired for two neighbouring CW/OA (CCW/OA) trimer units. MM simulations also imply that the + (or −) interdigitation mode is energetically unfavoured in neighbouring CW/OA (CCW/OA). Therefore, CW/OA trimers always follow the CW/OA units and interdigitate in +mode whereas CCW/OA trimers must follow CCW/OA units and adopt an interdigitation manner. As a result, two enantiomeric homochiral domains are formed by BIC at the OA/HOPG interface, just as revealed by STM. In the case of chiral R-OA or S-OA co-absorber, only CW/R-OA (or CCW/S-OA) trimer can form, as demonstrated in Fig. 5a . So, all trimers in the assembly possess the same handedness. These trimers may adopt either + or − interdigitation mode, as illustrated in Fig. 5b . The − (or +) interdigitation manner is preferred for CW/R-OA (or CCW/S-OA) trimer units considering the repulsion force and steric hindrance. Neighbouring CW/R-OA (or CCW/S-OA) trimers interdigitate to each other in the same − (or +) manner and form homochiral porous networks. Through this way, the induced CW (or CCW) homochirality in the BIC trimer units transfers and propagates to the 2D assembly and results in globally homochiral networks with CW (or CCW) handedness. The quantitative description of energy landscape during the induction and hierarchical amplification of homochirality is shown in Supplementary Fig. S5 . We want to point out that the chiral co-absorber induced homochiral assembly has distinct features. The chiral co-absorber 2-octanol is not only a chiral seed but also a building block in the assembly. The hexagonal network cannot exist in the absence of the co-absorber. As the interaction between chiral BIC trimers and 2-octanol is stereoselective and specific recognition exists between BIC trimers and co-adsorbed 2-octanol, the point chirality of the chiral co-absorber can determine the organization chirality of BIC trimer. In this sense, the assembly can be considered to be constructed by enantiopure supramolecules, that is, the ensemble of chiral aggregations of BIC trimer and co-absorber. On the basis of the above two points, it is apprehensible that either no hexagonal network forms or all the formed hexagonal networks possess the same handedness. In contrast, for the chiral sergeant controlled homochiral assembly of achiral soldier molecules, the sergeant molecules are structurally similar to soldier molecules. The homochirality of assembly stems from the cooperative interaction between ‘soldier molecules’ and ‘sergeant molecules’ and depends on the percentage of ‘sergeant molecules’ in the assembly [26] , [27] , [28] , [29] . The majority rules effect has been widely observed for 1D helical supramolecular polymer and analysed using theoretical models considering the penalty of helix reversal and mismatch [40] , [41] , [42] . For the 2D self-assembled hierarchical network presented here, it is believed the reversal and mismatch penalty is very high, considering the interactions between the assembly and the substrate as well as the strong intermolecular interactions. The possibility of chirality mismatch or reversion in an enantiomeric domain is very low as such high-energy structures can easily be avoided by dissociation of monomers back into the solution phase [43] . Therefore, the global surface chirality is believed to be dominated by the nucleation step [31] , [42] . Several molecules initially adsorbed on the solid surface from the solution determine the handedness of the assembly. MM simulations suggest that both the adsorption energy of S-OA and R-OA and the relative total energy for the formation of CCW/S-OA and CW/R-OA assembly are equal ( Table 1 ). It suggests enthalpies for the formation of two enantiomorphs of BIC assembly are the same, which is further confirmed by the comparable percentage of CW and CCW networks in the assembly when R-OA and S-OA present in the solution is equal. The bias for the CW and CCW assembly cannot be a result of the enthalpy but the entropy in the nucleation step. For an enatiomerically unbalanced solution of 2-octanol, there is always an entropy increasing driving force to reach equal amounts of S-OA and R-OA within the liquid phase to obtain the highest entropy. Therefore, the majority rather than the minority tends to adsorb on the solid surface from the solution to help increase the entropy of the solution phase (a rough derivation is shown in the Supplementary Methods ). As the reversal penalty and mismatch penalty for the BIC/2-OA co-assembly is high, the majority component can dictate the organization chirality of BIC network nuclei, and thus the formation of global homochiral network. The entropy-driven nonlinear chirality amplification has been proposed for 2D chirality organization of TA on Cu(110) in ultrahigh vacuum [31] . Intriguingly, recent theoretical modelling by Markvoort et al. [43] demonstrates that the nonlinear depletion of monomers into 1D helical supramolecular polymers occurs for the-majority-rule principle-based 1D helical assembly, involving distinct nucleation and growth processes. We believe the entropy effect is more pronounced for 2D assembly at the liquid/solid interface as the entropy driving force in the solution phase will barely vanish due to depletion of the majority chiral component to take part in the interface assembly. In addition, the preliminary results for the diluted majority rules experiment indicates that the nonlinear amplification strength is slightly decreased upon diluting the enantiomerically unbalanced solution with inert solvent. This result is consistent with the entropy-driven mechanism as (a) the entropy driving force is lowered upon dilution [43] ; (b) the chemical potential of chiral co-absorber in solution phase is lowered upon dilution and thus would rather stay in solution than adsorb on surface. In conclusion, we have presented the control of 2D global homochirality in molecular-assembled enantiomorphous networks of BIC by chiral co-absorber 2-octanol. Globally homochiral surfaces of the enantiomeric assembly of BIC are obtained using enantiopure chiral co-absorber 2-octanol or even mixed solution with as small as 5.2% ee in solution phase. The supramolecular recognition between chiral 2-octanol and chiral BIC trimers efficiently transfers the point chirality of co-absorber to the organization chirality of BIC aggregates, which then propagates to the 2D networks via hierarchical assembly. The majority rule principle is valid for the co-absorber-controlled homochiral assembly at the liquid/solid interface, which is driven by an entropy effect. Moreover, the global homochirality is memorized after the replacement of the chiral co-absorber by other achiral co-absorber. These results provide an alternative way towards globally homochiral surfaces and are beneficial for understanding the induction and amplification of homochirality in asymmetric heterogeneous catalysis and chiral separation. Experimental details BIC was home-synthesized [44] . For STM measurements, BIC was dissolved in solvent at a concentration of about 1 × 10 −5 M. To form a BIC assembly, 1.5 μl of such BIC solution was dropped onto a freshly cleaved HOPG (grade ZYB) surface. STM measurements were performed immediately at the liquid/solid interfaces using PicoSPM (Agilent Technologies). STM experiments were carried out at room temperature in constant-current mode using a mechanically cutting Pt/Ir wire (90/10) tip and shown without further processing. OA, S-OA and R-OA were purchased from Aldrich with purity of 99%. 1,16-hexadecanediol was from Aldrich with purity >95.0%. OB was from Tokyo chemical industry Co., LTD. All solvents were used directly. Statistical methods To calculate the area percentage of CW and CCW networks in the assembly, 5–10 samples were prepared for each measurement and at least 20 STM images with scan area of 100 × 100 nm 2 were recorded at different locations for each sample. The area of the CW and CCW networks in the STM images for one sample were summed up together, denoted with A CW and A CCW , respectively. The area percentage of CW and CCW network in the assembly (represented with R CW and R CCW , respectively) were calculated according to R CW = A CW /( A CCW + A CW ) and R CCW = A CCW /( A CCW + A CW ). Note that the area percentage given in the paper is an average value of several investigated samples. Theoretical simulations MM simulations were performed with the Tinker program using the MMFF force field [45] , [46] , [47] , [48] . The starting structures for MM simulations were built on the basis of STM images (see Supplementary Methods ). How to cite this article: Chen, T. et al. Globally homochiral assembly of two-dimensional molecular networks triggered by co-absorbers. Nat. Commun. 4:1389 doi: 10.1038/ncomms2403 (2013).